Direct observation of spin-forbidden transitions through the use of suitably polarized light The study of excited triplet states of a molecular system is a difficult task because accessing them involves forbidden transitions from the singlet ground state. Nevertheless, absorption spectra of many molecules present, at low energies, the weak fingerprint of these triplet states. At higher energies this information is usually masked by the intense signal of the singlet states. Here we show, for the specific case of the sulphur dioxide molecule, that the combined use of polarized light and molecular alignment can enhance the triplet part of the spectrum, even making it the only absorption process. In closed-shell systems, the spin-forbidden nature of the direct transition from the singlet electronic ground state (GS) to the excited triplet states prevents the direct study of the latter. Moreover, despite the fact that their weak signal can be observed in the low-energy region of the photoabsorption spectra of many compounds [1] , [2] , [3] , [4] , its analysis is hindered since, at higher energies, this information is usually masked by the intense signal from the allowed transition from the GS to singlet excited states. As a result, the characterization of the triplet states using the photoabsorption spectra is, in general, not possible over an extended energy range. The photoabsorption spectrum of the sulphur dioxide molecule (SO 2 ) in the near-ultraviolet range is a good example of the above situation. It presents two absorption bands, the so-called ‘forbidden band’ assigned to triplet electronic states [5] and for higher energies, the first allowed band assigned to singlet excited states [6] . Owing to its primordial relevance in various fields [7] , [8] , [9] , [10] , [11] , [12] , this molecule has been extensively investigated theoretically and experimentally over the past century. In this respect, a theoretical description of the ‘forbidden band’ has become available only recently [13] . However, as we show below, the approximations made in that study have led to an erroneous description of the underlying physical phenomenon. Here we demonstrate that the combination of molecular alignment and polarized light can improve our knowledge of the photoabsorption of the triplet states in molecular systems. As a key ingredient, we use an extended description of the vibronic GS of the molecule obtained by inclusion of its spin-orbit coupling (SOC) with triplet excited states, despite the large energy gap of ~3eV. As a result, we show that the singlet and triplet parts of the SO 2 spectrum originate from absorption of light with different polarization. We propose that this can be used advantageously to reduce or even dismiss the singlet part. We believe further that this situation is rather general and can be operative in other systems [1] , [2] , [3] , [4] such as O 3 , H 2 O, OCS and possibly in organic compounds as formaldehyde [14] . Description of the system In the near-ultraviolet range, the photoabsorption spectrum of SO 2 presents two absorption bands: (i) the so-called ‘forbidden band’ starting at 3.1 eV, assigned to triplet electronic states [5] , identified as the 3 B 1 and 3 A 2 states [15] , [16] ; and (ii) for energies greater than ~3.7 eV, the first allowed band, known as the Clements bands [6] , which is attributed to a transition to the coupled 1 B 1 / 1 A 2 singlet states [6] . A proper description of this band system (3.1–5.5 eV) of SO 2 requires the six lowest-lying electronic states, namely: three singlet states, the GS ( 1 A 1 ) and the first two excited states ( 1 B 1 and 1 A 2 ), as well as the three lowest triplet states ( 3 B 1 , 3 A 2 and 3 B 2 ). These are all the electronic states of SO 2 occurring in the energy range in question, the higher excited states being only involved in the second allowed band [17] , [18] (E>5.3 eV). The complexity of the system is enhanced by the presence of two symmetry-allowed conical intersections, see Fig. 1 , which result from displacement along the asymmetric vibration of the molecule, thus lowering its symmetry from C 2v to C s . The first one, between the 1 A 2 and 1 B 1 singlet states, has been accurately described in our recent work [19] . The second one, which involves the 3 B 1 and 3 A 2 triplet states of the same spin components M S , has been analysed here using our previous methodology [19] . In the following, C 2v labels will be used to discuss the different diabatic states. 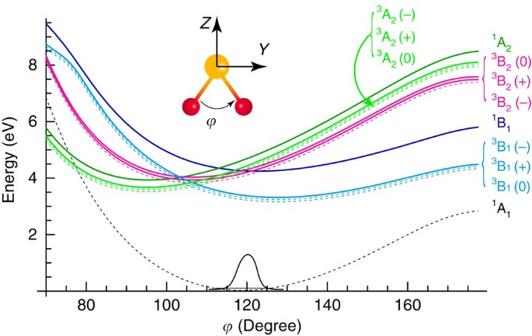Figure 1: Representation of the total system as treated herein. Cut of the potential energy surfaces of SO2along the bending angleφfor the 12 electronic states considered. Those belonging to the A′ or A′′ block of the Hamiltonian are represented as dashed and solid lines, respectively. The electronic GS of SO2, with its minimum at 119.8°, and equal S-O bond lengths of 1.448 Angstroms, is in black. The non-degenerate3B1(1B1) states are in light (dark) blue, while the light (dark) green lines represent the3A2(1A2) states and the magenta lines are the3B2states. Splitting between the different spin components is artificial, and given for a better graphical representation. In the cartoon the molecule and the Cartesian reference system used along this work are displayed. The molecule lies in the {y,z} plane, thexaxis being perpendicular to the figure. Figure 1: Representation of the total system as treated herein. Cut of the potential energy surfaces of SO 2 along the bending angle φ for the 12 electronic states considered. Those belonging to the A′ or A′′ block of the Hamiltonian are represented as dashed and solid lines, respectively. The electronic GS of SO 2 , with its minimum at 119.8°, and equal S-O bond lengths of 1.448 Angstroms, is in black. The non-degenerate 3 B 1 ( 1 B 1 ) states are in light (dark) blue, while the light (dark) green lines represent the 3 A 2 ( 1 A 2 ) states and the magenta lines are the 3 B 2 states. Splitting between the different spin components is artificial, and given for a better graphical representation. In the cartoon the molecule and the Cartesian reference system used along this work are displayed. The molecule lies in the { y , z } plane, the x axis being perpendicular to the figure. Full size image The inclusion of the SOC lifts the initial degeneracy of the different spin components of the triplet states ( M S =0, ±1). Then, introducing the symmetric (+) and asymmetric (−) combinations of states with M S =±1, we can write the Hamiltonian including the SOC interaction in block matrix form, with (i) one block of A′ symmetry, formed by the { 1 A 1 , 3 B 2 (−), 3 B 1 (+), 3 A 2 (+), 3 B 1 (0), 3 A 2 (0)} states; and (ii) one of A′′ symmetry collecting the { 1 B 1 , 1 A 2 , 3 B 2 (+), 3 B 2 (0), 3 B 1 (−), 3 A 2 (−)} ones. It should be noted that the A′ block includes the electronic GS ( 1 A 1 ), which lies about 3 eV below the other states in the block. Nature of the GS and photoexcitation The lowest GS vibrational states of the molecule were computed by Lanczos diagonalization of the full Hamiltonian of the A′ block—that is, including all the SOCs. Surprisingly, a small but non-negligible contribution from the triplet states (~10 −5 of 3 B 1 (0)) in the GS was found. Consequently, the vibronic GS should be written as where the index s runs over all the states of the A′ block. The electronic and nuclear coordinates are collected in r and R , respectively. The coefficients a s are the amplitudes, χ s ( R ) the vibrational wavefunctions on the electronic state s and φ s ( r ; R ) the corresponding electronic wavefunctions. This new vibrational state will be referred to as the perturbed vibrational GS to distinguish it from an unperturbed GS resulting from the 1 A 1 state alone. It is well known that in a photoexcitation event, the relative angle between the polarization of the incident light and the molecular frame can be of vital importance and induce different processes. If we assume the unperturbed vibrational GS of the molecule, the only allowed transition, within the considered state manifold, would take place between the 1 A 1 state and the 1 B 1 state, namely using x -polarized light (see Figs 1 and 2a for the axis system). As this is usually the only excitation considered in the absorption process, the polarization issue has never been addressed. 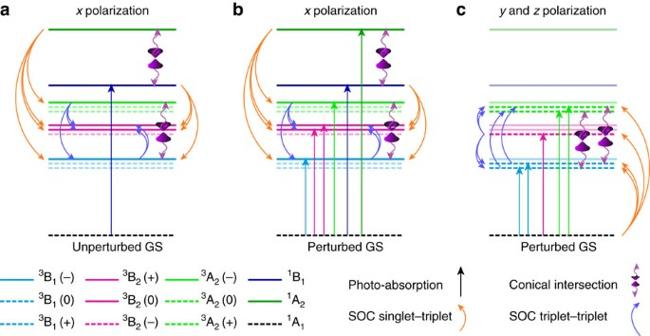Figure 2: Schematic representation of the different excitation mechanisms. Different mechanisms and couplings for the photoexcitation of SO2. We use the same colour code as inFig. 1.(a) Excitation from the unperturbed electronic GS of SO2. A direct photoabsorption (straight arrow) can take place from the GS to the1B1state withx-polarized light. The vibrational excited states are coupled through a conical intersection between the1B1and1A2states and SOC (blue and orange bent arrows) between all the different states of the A′ block.In addition, a conical intersection occurs between the states3B1and3A2. (b) The GS is perturbed by the SOC in the A′ block. More direct transitions could take place consideringx-polarized light, where the same coupling occurs as ina. (c) Direct transitions from the perturbed GS to the states of the A′ block withy- orz-polarized light. A direct excitation to the triplet A′ states takes place. Then, different couplings occur such as two conical intersections between the same spin components of the3B1and3A2states. Figure 2: Schematic representation of the different excitation mechanisms. Different mechanisms and couplings for the photoexcitation of SO 2 . We use the same colour code as in Fig. 1 . ( a ) Excitation from the unperturbed electronic GS of SO 2 . A direct photoabsorption (straight arrow) can take place from the GS to the 1 B 1 state with x -polarized light. The vibrational excited states are coupled through a conical intersection between the 1 B 1 and 1 A 2 states and SOC (blue and orange bent arrows) between all the different states of the A′ block.In addition, a conical intersection occurs between the states 3 B 1 and 3 A 2 . ( b ) The GS is perturbed by the SOC in the A′ block. More direct transitions could take place considering x -polarized light, where the same coupling occurs as in a . ( c ) Direct transitions from the perturbed GS to the states of the A′ block with y - or z -polarized light. A direct excitation to the triplet A′ states takes place. Then, different couplings occur such as two conical intersections between the same spin components of the 3 B 1 and 3 A 2 states. Full size image However, if the perturbed GS is considered, more transitions may take place depending on the polarization of the exciting radiation ( Fig. 2b,c ). Let be the total dipole moment operator and its Cartesian components. From symmetry considerations, it can be shown that induces transitions between states of the A′ and A′′ blocks, while provide transitions between states within the same symmetry block. Before the excitation, the initial wavefunction, perturbed or unperturbed, belongs to the A′ block, and thus the operators provide excitations within the A′ block only. The transition matrix can be written as: Here the initial wavefunction is projected, through the dipole moment operator, on a final state . The index μ runs over all the vibrational states of the excited electronic states, the vibrational state of being already included in its definition. Owing to the specific form of , the transition dipole moments as well as the dipole moments are involved in the excitation. More precisely, y -polarized excitation is dominated by the dipole moment (expectation value) promoting the triplet contribution of the perturbed GS to the corresponding triplet states, while z -polarized excitation is mostly governed by the transition dipole moment between different electronic states. Therefore, interferences between the different mechanisms are hardly noticeable. In addition, one should keep in mind that, as (i) we work in a diabatic basis and (ii) the SOC matrix elements are off-diagonal couplings, transitions between pure states of different spin multiplicities are forbidden. We shall consider now, from a formal perspective, the two possible coupling schemes (see Fig. 2 ) among the electronic states and their influences in the photoabsorption process, in particular, in relation to the ‘forbidden band’. The most straightforward picture results from the consideration of a SOC perturbation inducing an intersystem crossing between excited singlet and triplet states. Then, after a certain time after the excitation process, the wavepacket would start spreading over the remaining coupled states. An additional mechanism would arise if the SOC coupling would also induce a mixing of the singlet electronic GS and the triplet states, notwithstanding the energetic gap between them. The first explanation, responsible for the time-dependent population transfer between excited singlet and triplet states in the molecule, seems more plausible at first glance. This issue has been addressed in our recent work [20] , in which we have investigated the role of the SOC in the subgroup of A′ states after an excitation to the 1 B 1 diabatic state. This allowed transition dominates the excitation of the molecule in the 3.5- to 5.5-eV energy range and enables for the intersystem crossing to take place but does not account for the photoabsorption spectrum, the aspect that we are addressing here. The Clements bands [6] (3.7< E <5.5 eV) are governed by the allowed photoabsorption of the singlet states ( Fig. 3a ). They can be reproduced accurately when considering only the 1 B 1 and 1 A 2 states [19] , and the inclusion of the SOC ( Fig. 2a ) does not affect them significantly. As mentioned before, this part of the spectrum emerges from light polarization perpendicular to the molecular plane. This is not the case of the ‘forbidden band’, which exhibits an opposite dependence on the light polarization. This emanates from the different possible mechanisms of excitation of the perturbed GS (see Fig. 2b,c ). 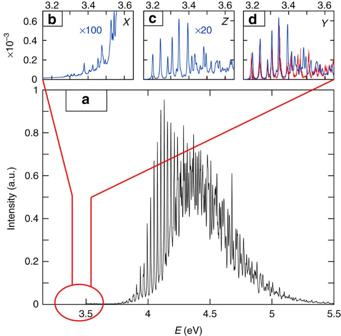Figure 3: Photoabsorption spectra depending on the light polarization. Theoretical photoabsorption spectra obtained from the Fourier transform of the autocorrelation function from a wavepacket propagation for 1 ps (except forx-polarization for which we used diagonalization due to the weakness of the spectrum in comparison to the singlet one (a). A damping function of 300 fs is used to reproduce the experimental linewidth. (a) Full spectrum in the range 3.15–5.5 eV, with the Clements bands resulting from the singlet states (E>3.7 eV). Framesb–dpresent the spectra of the triplet states (three orders of magnitude lower in intensity) after alignment of the molecules and forx-,y-andz-polarized light, respectively. The theoretical spectrum (blue line) ofdis superimposed with the experimental spectrum (red line) of Vandaeleet al.4, showing very good agreement. Figure 3: Photoabsorption spectra depending on the light polarization. Theoretical photoabsorption spectra obtained from the Fourier transform of the autocorrelation function from a wavepacket propagation for 1 ps (except for x -polarization for which we used diagonalization due to the weakness of the spectrum in comparison to the singlet one ( a ). A damping function of 300 fs is used to reproduce the experimental linewidth. ( a ) Full spectrum in the range 3.15–5.5 eV, with the Clements bands resulting from the singlet states ( E >3.7 eV). Frames b – d present the spectra of the triplet states (three orders of magnitude lower in intensity) after alignment of the molecules and for x- , y- and z -polarized light, respectively. The theoretical spectrum (blue line) of d is superimposed with the experimental spectrum (red line) of Vandaele et al. [4] , showing very good agreement. Full size image For x -polarized light, the spectrum ( Fig. 3b ) exhibits features in the low-energy region ( E <3.5 eV), which are two orders of magnitude smaller than the experimental ones, and show a totally different vibrational progression. This strong discrepancy refutes the idea that it arises from the intersystem crossing between these states, as recently proposed [13] . There, a SOC between the 1 B 1 and 3 B 1 states was implicitly considered, despite being forbidden by symmetry. Without this incorrect assumption, one cannot recover the experimental spectrum anymore. If, on the other hand, we consider the excitation of the perturbed GS using y - or z -polarized radiation ( Fig. 2c ), we obtain the characteristic part of the triplet spectrum ( Fig. 3c,d ) in excellent agreement with experiment [4] , both regarding the spectral intensity distribution within the triplet energy range and the overall intensity (for the y -polarized excitation) relative to the singlet spectrum. This demonstrates that the perturbation occurring on the GS vibrational wavefunction due to the SOC in the A′ manifold of states is mandatory to interpret the experimental spectrum. To clarify the role of the SOC in the different manifolds of states (A′ or A′′), we have performed simulations where we either included the SOC in the excited states with an unperturbed GS wavefunction ( Fig. 2a ) or neglected the SOC in the excited states keeping the perturbed wavefunction for the GS. In the first case, the x -polarized spectrum resembles the one in Fig. 3b but, as the y and z excitations are forbidden by symmetry, it cannot alone match the experimental triplet spectrum. In the second case, the y - and z -polarized spectra are not affected, and the x -polarized spectrum presents almost no features below 3.55 eV. Therefore, it can be concluded that the triplet spectrum of SO 2 can be attributed exclusively to the perturbed GS wavefunction, resulting from the SOC within the A′ state manifold. The interesting point that should be stressed is that the two mechanisms present an antagonistic dependence on the polarization of light, in turn, providing us with an experimental way to disentangle their contribution. To the best of our knowledge, the proposed mechanism has never been suggested before in this context and provides a new way to depict the photoexcitation of SO 2 . It is reminiscent of what is reported in the spectroscopy of certain transition metal complexes, for which a strong SOC induces a large mixing for both ground and excited states and permits the observation of bands otherwise forbidden [21] . In contrast, in SO 2 , the GS mixing is the only relevant aspect for the triplet absorption spectrum. It should be mentioned that, in the context of the radiative lifetime of formaldehyde, Phillips and Davidson [14] pointed out in their ab initio study a similar mixing scheme between distant electronic states (energetic gap ~1 eV). The study was limited to the computation of the transition dipole moment, and the effect on the vibronic states of the molecule was not included. The experimental information of the triplet states in this system mainly derives from the study of this forbidden band but, as demonstrated, this part of the spectrum is uncorrelated to the six other relevant states. Therefore, no information concerning the SOC between the excited singlet and triplet A′ states can be extracted from these measurements. Furthermore, we can explain the absence of experimental evidence of the 3 B 2 state in the spectrum, despite its theoretical prediction [22] . It proceeds from an extremely low weight (10 −11 ) in the perturbed GS due to a particularly weak SOC with the 1 A 1 state; hence, only the 3 B 1 and 3 A 2 states play a role in the energy range of Fig. 3b,c . The importance of the intersystem crossings for the time-dependent dynamics in the A′ states [20] is due to the higher energy range treated in that work. As already mentioned, for energies greater than 3.6 eV the triplet contribution is masked by the intense signal from the singlet states ( Fig. 3a ). To overcome this, we propose the use of the strong polarization dependence to suppress the singlet part of the Clements bands, thus revealing a new part of the triplet spectrum. To this end, the SO 2 molecules should be oriented before excitation with linearly polarized UV light. The orientation could be achieved, for instance, through impulsive laser excitation [23] , [24] as it has been already successfully demonstrated for SO 2 (refs 25 , 26 ). In Fig. 4 , we show the signal from the y -polarization, which is strongly damped at energies higher than 4 eV, while the z -polarized excitation exhibits a stronger absorption for energies between 3.7 and 5 eV. This new part of the spectrum, never observed or predicted before, results mainly from the excitation from the 3 B 1 (0) component of the GS wavefunction to the excited 3 A 2 (0) state via the transition dipole moment operator along the z axis. 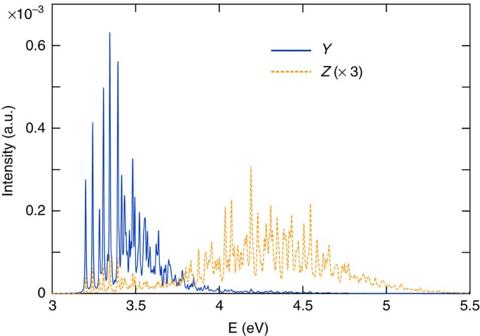Figure 4: Photoabsorption in the 3–5.5 eV range. Theoretical photoabsorption spectra (same asFig. 3b,c) depicted from 3 to 5.5 eV—that is, in the energy range of the Clements bands. In the full blue line the spectrum is shown resulting from ay-polarized excitation and in the dashed orange line as resulting fromz-polarized excitation. For better visibility, thez-polarized spectrum has been multiplied by a factor 3. Figure 4: Photoabsorption in the 3–5.5 eV range. Theoretical photoabsorption spectra (same as Fig. 3b,c ) depicted from 3 to 5.5 eV—that is, in the energy range of the Clements bands. In the full blue line the spectrum is shown resulting from a y -polarized excitation and in the dashed orange line as resulting from z -polarized excitation. For better visibility, the z -polarized spectrum has been multiplied by a factor 3. Full size image In conclusion, we have shown that the polarization of the excitation has a crucial impact on the photoabsorption spectrum of SO 2 , offering us the possibility to decouple the contributions of the A′ and A′′ sub-systems. Exclusively preparing the A′ system requires aligning the molecules at least in a plane before in- or out-of-plane linearly polarized UV excitation. Even though a perfect alignment for the whole sample is not realistic, the antagonistic effect of the polarization on the A′ and A′′ sub-systems, demonstrated in this work ( Fig. 3b,c ), makes it possible to elucidate the different mechanisms and obtain the corresponding spectra. The experimental probe/test of the role played by the perturbed GS relies on the fact that the triplet part of the spectrum shows up at lower energies than the singlet signal. For an anisotropic distribution of the molecules in the sample, incident polarized light will modulate the relative intensity between the singlet and triplet parts of the spectrum. We emphasize that our reasoning is not limited to SO 2 but is relevant to many other systems where a symmetry element is present, allowing one to distinguish experimentally the SOC effects involving the GS (here A′ symmetry) from the SOC within the excited-state manifold (here A′ symmetry). Thus, it may apply to any triatomic molecule and also to larger systems where, for a given dynamic process, a plane of symmetry (or similar) plays a role. Quantum chemistry calculations The potential energy surfaces have been calculated at the MRCI level of theory based on a CAS-SCF electronic wavefunction using an active space comprising 18 electrons in 12 orbitals and a cc-pVTZ basis set. For the potential energy surface of each state, at least 16,000 points at different geometries have been computed. The SOC matrix elements have been obtained from the Breit–Pauli operator for 2,000 different geometries to take into account their coordinate dependence. At these same geometries, we have also computed the dipole moment and transition dipole moments at the MRCI level. The relevant SOC (absolute values) between the GS and the excited states of the A' block in the region of the C 2v minimum are ~145 cm −1 for 3 B 1 (0), ~50 cm −1 for 3 A 2 (+), ~0.5 cm −1 for 3 B 2 (−) and vanishing by symmetry for 3 B 1 (+) and 3 A 2 (0). The MOLPRO [27] programme suite was employed throughout. Perturbed GS The perturbed GS is obtained using the Lanczos diagonalization algorithm on the full A′ block—that is, the 1 A 1 , 3 B 2 (−), 3 B 1 (+), 3 A 2 (+), 3 B 1 (0), 3 A 2 (0) plus all the SOCs between them. The lowest eigenfunction shows a mixing of the wavefunction of the 1 A 1 state (0.99997157), the 3 B 1 (0) state (2.63598819 × 10 −5 ) and the 3 A 2 (+) state (1.96550847 × 10 −6 ), while the other states contribute to less than 10 −8 . Initial wavefunction The initial wavefunction, for the propagation or the projection on the eigenstates during the diagonalization, is computed by applying the corresponding matrix elements of the total dipole moment operator for the respective transitions occurring between the A′ and A′′ blocks for an x -polarized excitation and inside the A′ block for y - and z -polarized ones. Spectra The photoabsorption spectra are computed in two different ways, both performed with the Heidelberg MCTDH software package [28] using a discrete variable representation to expand the wavefunctions. (i) The initial wavefunction is propagated during 1 ps under the action the A′ or A′′ block Hamiltonian and used to compute the autocorrelation function. The Fourier transform of the latter leads to the absorption spectra presented in this work. (ii) For the x -polarization case, due to the extreme weakness of the triplet contribution compared with the allowed Clements bands, computed in (i), the full A′ block, including all the SOCs between these states, has been diagonalized. The projection of the initial wavefunction on the obtained eigenstates leads to the spectrum, after a convolution using a Lorentzian function to mimic the experimental resolution. In order to compare our results with experiment, we have matched together the intensities of the singlet spectra and then directly compared with the triplet spectra without further adjustment. How to cite this article: Lévêque, C. et al. Direct observation of spin-forbidden transitions through the use of suitably polarized light. Nat. Commun. 5:4126 doi: 10.1038/ncomms5126 (2014).